Chemical processes in the deep interior of Uranus The unusual magnetic fields of the planets Uranus and Neptune represent important observables for constraining and developing deep interior models. Models suggests that the unusual non-dipolar and non-axial magnetic fields of these planets originate from a thin convective and conducting shell of material around a stably stratified fluid core. Here, we present an experimental and computational study of the physical properties of a fluid representative of the interior of Uranus and Neptune. Our electrical conductivity results confirm that the core cannot be well mixed if it is to generate non-axisymmetric magnetic fields. The molecular dynamics simulations highlight the importance of chemistry on the properties of this complex mixture, including the formation of large clusters of carbon and nitrogen and a possible mechanism for a compositional gradient, which may lead to a stably stratified core. The non-axisymmetric nature of the Uranian and Neptunian magnetic fields creates specific demands on magnetohydrodynamic models of Uranus and Neptune. Stanley and Bloxham [1] , [2] successfully produced planetary models with non-axisymmetric magnetic fields generated within a thin fluid shell. The specific properties of the inner core for these models have a key role in whether non-axisymmetric magnetic fields are generated. Both solid non-conducting inner cores or stably stratified fluid cores (conducting or non-conducting) lead to non-axisymmetric magnetic fields similar to Uranian and Neptunian magnetic fields. These planetary models depend on knowing the physical properties of the fluids that make up the interior of planet such as electrical conductivity, viscosity and structure of the fluids. In the case of Uranus and Neptune, the major components of the interior of the planets are thought to resemble mixtures of water, methane and ammonia. Unlike the hydrogen/helium dominated Jovian planets, complex chemical processes are expected for such mixtures of molecular fluids at deep planetary conditions, several 100 GPa and several 1,000 K. Do these chemical processes create conditions within Uranus and Neptune favourable for the formation of the unique interior structures predicted by the current models of the non-axisymmetric magnetic fields? Advances in experimental and computational techniques allow for the improved determination of the physical properties of materials under planetary conditions. Improved estimations for properties such as electrical conductivity and viscosity (Reynolds number) are needed to model the behaviour of such planets. For example, the electrical conductivity profile used most dynamo models is assumed to be constant below a certain depth based on previous experimental studies of water at high pressures [3] . Although there exists a vast gap between planetary and laboratory timescales, important insight can be gained. Here, we explore the properties of a synthetic Uranus (SU) mixture with chemical abundance ratios of H:O:C:N=28:7:4:1. The SU mixture is a single-phase mixture of water, ammonia and isopropanol that is liquid at atmospheric pressure and room temperature and has an atomic composition representative of icy planets. Some aspects of the SU mixture such as equation of state Hugoniot (P-V-E) data, temperatures and electrical conductivities of SU have been measured under single-shock compression up to 70 GPa (0.7 Mbar) (refs 5 , 6 , 7 ) and under double-shock compression up to 200 GPa (ref. 7 ). These single-shock experiments did not reach pressures comparable to the deep interior, whereas double-shock experiments did not measure the electrical conductivity and the temperatures reached are above those expected on the planetary adiabat. This work is focused on studying the properties of the SU mixture at conditions corresponding to the deep interior of Uranus and Neptune. Using a reverberating shock, we can reach states closer to those on the planetary adiabat and reach P and T conditions much deeper into the planet. Electrical conductivity measurements are particularly useful because they provide direct input into dynamo models and such measurements are useful probes of chemical processes. We examine the structure of the complex fluid and the associated chemistry using first-principles molecular dynamics (FPMD) to understand possible mechanisms for generating predicted interior structures of Uranus and Neptune. We show that the electrical conductivity of the SU mixture increases monotonically with pressure and scales with that of water as a function of density. The inclusion of carbon and nitrogen atoms in the SU mixture inhibit the formation of the superionic phase of water. The C–C and C–N bond lifetimes are shown to be longer lived than other bonds and may indicate clustering. The clustering of C and N atoms would lead to a segregation of the fluid and the formation of a stratified core with a low conductivity consistent with the current models. Electrical conductivity experiments The electrical conductivity of SU was measured from 74 to 191 GPa as described in Methods. 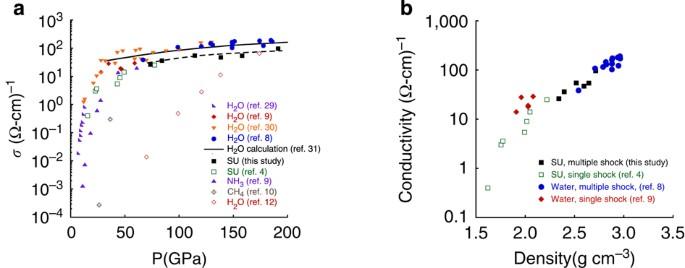Figure 1: The electrical conductivity of water and SU plotted as a function of pressure and density. (a) The water data of Haman and Linton29and Mitchell and Nellis9and the SU data of Nelliset al.4are single-shock data, whereas the water data of Chauet al.8are from multiple-shock data. Also shown for comparison purposes are the single-shock data for methane10and ammonia9. The dashed line is a guide for the eyes. (b) the electrical conductivity of water and SU plotted as a function of density. Figure 1a shows the electrical conductivity data of SU as a function of pressure. For a useful comparison, the electrical conductivity data for individual constituents [8] , [9] , [10] that make up the interior of Uranus (water, ammonia and methane) are also shown in Figure 1 . The previous single-shock data on SU showed a five order of magnitude increase in electrical conductivity from ambient to about 50 GPa and reached the value of ~20 (Ω-cm) −1 The higher pressure data in this work shows that the electrical conductivity of SU continues to increase monotonically by a of factor 3 between 50 to 191 GPa. The rapid increase of the electrical conductivity to ~30 GPa followed by a slower increase to very high pressures is very similar to the behaviour observed in water [8] although the magnitude of the electrical conductivity in SU is approximately a half that of water. Figure 1: The electrical conductivity of water and SU plotted as a function of pressure and density. ( a ) The water data of Haman and Linton [29] and Mitchell and Nellis [9] and the SU data of Nellis et al . [4] are single-shock data, whereas the water data of Chau et al . [8] are from multiple-shock data. Also shown for comparison purposes are the single-shock data for methane [10] and ammonia [9] . The dashed line is a guide for the eyes. ( b ) the electrical conductivity of water and SU plotted as a function of density. Full size image The previous experiments on SU [4] were performed using a single-shock technique that reaches a higher temperature for a given final pressure as compared with the multiple-shock technique used in this study. A comparison of the highest pressure data from the single-shock experiments and the lowest pressure data from this study show the same electrical conductivity. This suggests that the electrical conductivity is nearly temperature independent below ~75 GPa. The data for ammonia and methane are limited to single-shock experiments up to 30 GPa. Ammonia behaves much like water below 30 GPa with a slightly lower conductivity. In contrast, methane is a poorer conductor than water, ammonia and SU below 150 GPa. The conductivity of methane only becomes comparable to that of water, ammonia and SU above 150 GPa (unpublished). In general, the body of experimental data on planetary ice materials either as pure compounds or in mixture suggest that the electrical conductivity will increase with pressure and temperature, eventually becoming metallic. Thus, as one approaches the core of the planet the conductivity will increase monotonically if there is not a compositional gradient. FPMD simulations The electrical conductivity experiments give insight into the bulk behaviour of the SU mixture, but do not shed any light into local chemical structure of the fluid. Experimental probes of the local structure at the conditions of the deep interior of Uranus and Neptune remain elusive. To progress further, we examined the possible local structure of the SU fluid and the chemistry using FPMD. 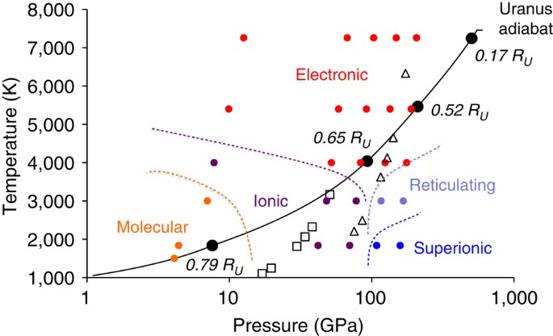Figure 2: P–T space diagram of synthetic Uranus. The filled circles are from the FPMD calculations. Opened squares are the measured P and T after the initial shock. Opened triangles are the estimated P and T reached in the reverberating shock. The colours represent different phases of the fluid. The black line is the planetary adiabat of Uranus (personal communication). Figure 2 summarizes the pressure and temperature space that was explored with FPMD. This phase space is partitioned into several regions highlighting certain characteristics of the SU mixture.The solid black line is a planetary adiabat of Uranus (personal communication from W. Hubbard) that represents expected states within Uranus. Figure 2: P–T space diagram of synthetic Uranus. The filled circles are from the FPMD calculations. Opened squares are the measured P and T after the initial shock. Opened triangles are the estimated P and T reached in the reverberating shock. The colours represent different phases of the fluid. The black line is the planetary adiabat of Uranus (personal communication). Full size image We identify five regions: molecular, ionic, superionic, reticulating and electronic. In the molecular phase, bond lifetimes for bonds involving hydrogen are long and charge carriers are molecular units. In addition, in this phase the hydrogen atoms have essentially the same diffusivity as the oxygen atoms. In the ionic phase, bond lifetimes for bonds involving hydrogen are shorter and the hydrogen atoms diffuse at least twice as fast as any other atom. In the superionic phase, hydrogens are the only carriers. The larger atoms are essentially frozen in a disordered state, and the system has a band gap. There is a sharp decrease in the electronic conductivity of SU at 1,873 K. The superionic phase forms at a much lower temperature than in pure water. In the reticulating phase, the larger atoms have diffusivity coefficients typical of fluids (~5×10 −5 cm 2 s −1 ), but bond lifetimes for C–C and C–N bonds are long and large organic molecules/network can form (hence the name reticulating). In the electronic phase, the electronic conductivity is the dominant part of the total conductivity and bond lifetimes are very short. In addition to useful transport properties such as diffusivity, conductivity and viscosity, the analysis of the molecular dynamics (MD) trajectories through the use of correlation functions such as the bond auto-correlation function (BACF) can shed light on the complex chemistry that is occurring in the SU mixture under these pressure and temperature conditions. The BACF β ( t ) is defined as where the bond vector B is a byte vector with value of 1 for each bond of a certain type within a cutoff distance and 0 otherwise. This correlation function describes the average duration of a bond between two atoms. The decay timescale (or the bond lifetime) is not strongly dependent on the chosen bond cutoff. We use 1.7A ˚ for bonds between large atoms, 1.3A ˚ for bonds between large atoms and hydrogen and 0.9A ˚ for hydrogen–hydrogen bonds. 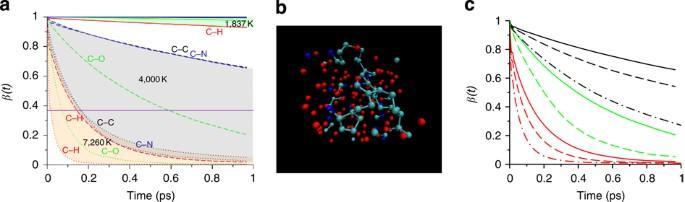Figure 3: Bond auto-correlation functions (BACF) of H2O, CH4, mixture of H2O–CH4and SU. (a) BACF for four type of bond: C–C (black), C–N (blue), C–O (green) and C–H (red) for different temperatures (1,837 K: solid lines green shading, 4,000 K: dashed lines grey shading and 7,260 K: dotted lines orange shading) at a density of 3 g cm−3(this corresponds to a pressures of 160, 176 and 200 GPa, respectively); (b) A snapshot of the molecular dynamics simulation at a density of 3 g cm−3at 4,000 K. This corresponds to the reticulating phase. Carbon atoms are light blue, oxygens are red, nitrogens are blue and hydrogens have been masked to highlight the scale of the carbon network; (c) BACF of different mixtures at 4,000 K and 176 GPa. Black denote C–C bonds, green denote C–O bonds and red denote C–H bonds. The solid lines represent the synthetic Uranus, the dashed line represent a water–methane mixture and the dot dashed line represents pure methane. In Figure 3a , we present the BACF of the SU mixture for four types of bond: C–C (black), C–H (red), C–O (green) and C–N (blue) for different temperatures (1,837, 4,000 and 7,260 K) at a density of 3 g cm −3 (this corresponds to pressures of 160, 176 and 200 GPa, respectively). At lower temperature (1,837 K, green shaded area, solid lines), the bond lifetimes for C–C, C–N, C–O and C–H are all quite long. At very high temperature (7,260 K, orange shaded area, dotted lines) the bond lifetimes for all three type of bonds are very short, smaller than 0.2 ps (time for which the correlation function is equal to 1/e ( Fig. 3a ). At intermediate temperature (4,000 K, grey shaded area, dashed lines), the bond lifetimes have very different values depending on the type of bond: C–H bonds are very short lived, C–O bonds last about three times longer and C–C and C–N are at least an order of magnitude longer. This is correlated with the presence of large organic molecules in our first-principles simulations of the planetary fluid and determines a phase of the synthetic Uranus mixture, we call this as the reticulating phase. Figure 3: Bond auto-correlation functions (BACF) of H 2 O, CH 4 , mixture of H 2 O–CH 4 and SU. ( a ) BACF for four type of bond: C–C (black), C–N (blue), C–O (green) and C–H (red) for different temperatures (1,837 K: solid lines green shading, 4,000 K: dashed lines grey shading and 7,260 K: dotted lines orange shading) at a density of 3 g cm −3 (this corresponds to a pressures of 160, 176 and 200 GPa, respectively); ( b ) A snapshot of the molecular dynamics simulation at a density of 3 g cm −3 at 4,000 K. This corresponds to the reticulating phase. Carbon atoms are light blue, oxygens are red, nitrogens are blue and hydrogens have been masked to highlight the scale of the carbon network; ( c ) BACF of different mixtures at 4,000 K and 176 GPa. Black denote C–C bonds, green denote C–O bonds and red denote C–H bonds. The solid lines represent the synthetic Uranus, the dashed line represent a water–methane mixture and the dot dashed line represents pure methane. Full size image The pressure dependence of the electrical conductivity of SU is very much similar to that of water and ammonia where there is a sharp rise in conductivity at low pressures followed by a plateau above 30 GPa (refs 8 , 9 ). The low pressure conductivity is dominated by conduction via H + ions that have an effective mean free path comparable to the nearest neighbour distance and travel at thermal velocity. The interpretation is that below 30 GPa, the molecular bonds are being broken generating an increasing population of H + charge carriers. Based on this picture one can apply the Drude model to the conductivity in which one H + ion per molecule is available as a charge carrier, one finds the electrical conductivity to be of order 30 (Ω-cm) −1 roughly in agreement with the data. It is interesting that if one applies this picture to increasing pressure, a decrease in conductivity would result because of the shortening of the mean free path, which is contrary to the current experimental data that show a monotonic increase with pressure. The further increase in electrical conductivity is due to the gradual onset of electronic conduction. The temperature independence of the electrical conductivity ≤74 GPa is consistent with ionic dominated conduction. At higher pressures, electronic conduction will become more pronounced and eventually dominate the ionic contribution. Electronic conduction at higher pressures is expected to be hydrogen-like wherein the electrical conductivity is thermally activated (semi-conductor-like) and temperature dependent with an energy gap that closes with pressure [11] . The electrical conductivity would become metallic-like on the closing of the gap. The transition from ionic dominated to electronic dominated conduction is smooth and continuous, and not accompanied by any observable discontinuities. In laser shock experiments on water, metallic-like conductivity was reported at very high pressures and different temperatures from this study [12] , [13] . The laser experiments are only sensitive to the electronic part of the conductivity and are lower than our reported conductivity, which includes both the ionic and electronic contributions. As the pressure and temperature increases, the electronic contribution to the conductivity will increase and eventually dominate the ionic contribution. The onset of electronic conduction also leads to electronic contributions to the specific heat and thermal conductivity. We do not have estimates of these contributions but their effect on the thermal profiles of the planet's interior cannot be neglected. The similarity of the pressure dependence of the electrical conductivity of SU and water is not surprising, as SU is mostly composed of water. The fact that the conductivity versus pressure relation for SU appears to be shifted down from that of water by a factor of two, suggested a possible scaling of the electrical conductivity. The conductivity of water and SU are plotted in Figure 1b as a function of density. As a function of density, the electrical conductivity of water and SU are identical. The density is a measure of the next nearest neighbour distance or effectively the scattering distance for an ion. This makes sense for the ionic conductivity in which the ions have a mean free path that is approximately the next nearest neighbour spacing. It is unclear why this works for the electronic contribution. Ignoring the specific effects of chemistry, the fluid ice layers of Uranus and Neptune can be effectively modelled by density-scaled water. It is instructive to compare the SU mixture to simpler systems, such as water, methane, and water–methane mixtures (1:1), in particular, in the reticulating phase (4,000 K and 176 GPa). In the region denoted as the reticulating phase in Figure 2 (~4,000 K and 176 GPa), FPMD simulations of pure water predict it to be in the superionic phase [14] with a solid oxygen lattice. This is no longer the case in FPMD simulations of mixtures of water–methane or SU, in which the addition of carbon promotes the diffusion of oxygen atoms. Such a change in the location of phase lines in mixtures compared with the pure components is to be expected, and we recover a 'superionic' phase at the same density (3 g cm −3 ) but at much lower temperature (1,837 K), in which the larger atoms are essentially frozen (diffusion coefficient of ~10 −6 cm 2 s −1 ), whereas the hydrogen (deuterium) are still fluid (diffusion coefficient of 7.7×10 −5 cm 2 s −1 ). However, at this scale no long-range order is apparent in the simulations. From the simulations we find that under these extreme conditions of pressure and temperature, molecules dissociate and react at very rapid rates. In the reticulating phase, as the bond lifetime of C–C and C–N bonds is much longer than other type of bonds, the large organic molecules observed in the simulation may be the first stage of growing clusters (containing mostly carbon but also nitrogen). The dissociation of pure methane has been suggested to lead to the precipitation of the carbon in the form of diamond [15] . But, in the case of the shock recovery experiments and the static high pressure experiments on methane, the presence of aggregated carbon is confirmed only on release to ambient conditions and does not indicate the state of the carbon at high pressure and temperatures. Under the influence of gravity, these small clusters (which are denser than the surrounding fluid) are expected to sink deeper into the core of the planet and constitute a large source of (gravitational) energy that will be converted into thermal energy deeper in the planet. If the clusters forming in the reticulating phase of the SU mixture, indeed, lead to segregation and precipitation of the carbon and nitrogen content of the mixture, one would go from a fluid highly conducting mixture to an essentially solid superionic water fraction with a rather low conductivity (only ionic through proton hopping with no electronic component), whereas carbon would be in the diamond phase, which has essentially no conductivity. This would then support a stratified core with very low conductivity in line with the models of Stanley and Bloxham [1] . To highlight the role of water on the carbon chemistry in the reticulating part of the P–T space, we compare the BACF for C–C and C–H bonds in methane, water–methane (1:1) and SU (which is 1.75:1 O to C ratio) at 4,000 K and 176 GPa (see Fig. 3c ). We find that the C–C bonds have a longer lifetime for water-richer mixtures. This suggests that the water-rich SU mixture favours the formation of larger carbon network or clusters than the water–methane (1:1) mixture. This tendency could also be due to the presence of N. In the reticulating phase, although the SU mixture is still fluid, because of the C–C and C–N bonding and the formation of large networks, its viscosity is expected to be quite different from that of the higher temperature fluid. 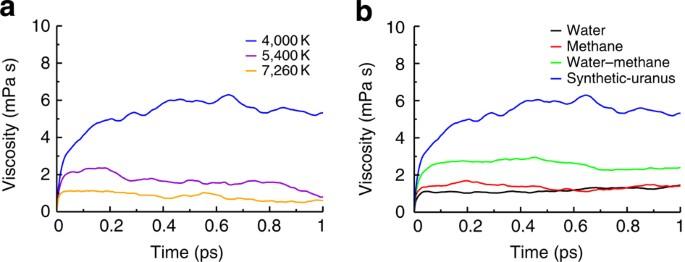Figure 4: The calulated viscocity of synthetic Uranus and other mixtures. (a) Calculated viscosity of the synthetic Uranus mixture as a function of temperature. The viscosity is six times higher at 4,000 K than at 7,260 K. (b) Calculated viscosity of different mixtures at 4,000 K and 176 GPa. At 4,000 K and 176 GPa, the viscosity of the SU mixture is higher than that of the other fluids considered such as methane and water–methane (1:1). The calculated viscosity for SU and other mixtures are shown in Figure 4 . We find that the viscosity is indeed six times higher at 4,000 K than at 7,260 K. Moreover, at 4,000 K and 176 GPa, the viscosity of the SU mixture is higher than that of the other fluids considered such as methane and water–methane (1:1). This is consistent with the results from the BACF in that the carbon clusters are more stable in the SU mixture. Figure 4: The calulated viscocity of synthetic Uranus and other mixtures. ( a ) Calculated viscosity of the synthetic Uranus mixture as a function of temperature. The viscosity is six times higher at 4,000 K than at 7,260 K. ( b ) Calculated viscosity of different mixtures at 4,000 K and 176 GPa. At 4,000 K and 176 GPa, the viscosity of the SU mixture is higher than that of the other fluids considered such as methane and water–methane (1:1). Full size image In applying shock compression data to planetary problems, the vast difference between laboratory and planetary timescales needs to be addressed. On the experimental timescale of hundreds of nanoseconds, we expect that the number of particle collisions is sufficiently high for thermal equilibrium to be achieved. However, the ice fluid at planetary pressures and temperatures is expected to be a dissociated fluid and it becomes unclear over planetary timescales whether the effects of gravity and other forces such as convection lead to chemical separation of the dissociated products or if rough chemical balance is maintained. Shock recovery experiments on a variety of hydrocarbons typically show irreversible dissociation of the hydrocarbons and the formation of small amorphous carbon particles. In the case of methane, our preliminary data suggest this process occurs within hundreds of nanoseconds or less. This suggests that any methane within planetary interiors would likely have dissociated and precipitated out as some form of carbon. The situation is less clear for the dissociation products of water and ammonia, but from the simulation, it is likely that the nitrogen is incorporated in the carbon clusters. Any separation and segregation of dissociated products would support the possibility of a stratified inner core for Uranus and Neptune. Electrical conductivity measurement The experimental technique is the same one used in previous studies of water [8] . Dynamic pressure was generated with a two-stage light-gas gun [4] using a reverberating shock wave. The electrical conductivity of the SU sample was measured as a function of time. In these experiments, the final pressure in the SU sample ranged from 74 to 191 GPa. These final pressures are equivalent to ~0.675 to 0.5 Uranus radii and ~0.7 to 0.6 Neptune radii based on the density-radii calculations of Hubbard [7] . The final shock pressure was determined by impedance matching [11] whereas the density of SU was calculated using the one-dimensional hydrodynamics codes ONEDEE and KOWIN [16] , [17] . For the equation of state of SU, we used the experimentally measured Hugoniot data [4] and a simple Grüneisen model. We estimated the temperature by assuming the first shock temperature is 60% of the final temperature and the first shock temperature was determined by previous measurements of shock temperature versus pressure [5] . This is an empirical estimate based on the fact that a reverberating shock wave is composed of a strong first shock and a series of weak shocks. The bulk of the temperature is generated on the first and second shocks [18] . The measured values of electrical conductivities and pressures, and the estimated volumes and temperatures are given in Table 1 . Table 1 Experimental data for SU obtained using a two-stage light-gas gun. Full size table MD simulations The calculations were performed with VASP [19] , [20] , [21] , [22] using a 600 eV energy cutoff, a time step of 0.2418 fs, the Perdew-Burke-Ernzerhof (PBE) [23] , [24] exchange-correlation functional, projector augmented wave method (PAW) pseudopotentials [25] , [26] and Nosé-hoover thermostat [27] , [28] . The states were occupied according to a Fermi distribution at the system's temperature. The MD was run at the gamma point and the electric conductivity were evaluated using the k-point. How to cite this article: Chau, R. et al . Chemical processes in the deep interior of Uranus. Nat. Commun. 2:203 doi: 10.1038/ncomms1198 (2011).